Terahertz single conductance quantum and topological phase transitions in topological insulator Bi2Se3ultrathin films Strong spin-orbit interaction and time-reversal symmetry in topological insulators generate novel quantum states called topological surface states. Their study provides unique opportunities to explore exotic phenomena such as spin Hall effects and topological phase transitions, relevant to the development of quantum devices for spintronics and quantum computation. Although ultrahigh-vacuum surface probes can identify individual topological surface states, standard electrical and optical experiments have so far been hampered by the interference of bulk and quantum well states. Here, with terahertz time-domain spectroscopy of ultrathin Bi 2 Se 3 films, we give evidence for topological phase transitions, a single conductance quantum per topological surface state, and a quantized terahertz absorbance of 2.9% (four times the fine structure constant). Our experiment demonstrates the feasibility to isolate, detect and manipulate topological surface states in the ambient at room temperature for future fundamental research on the novel physics of topological insulators and their practical applications. Robust topological surface states (TSSs) on topological insulators (TIs), such as Bi 2 Se 3 , Bi 2 Te 3 and Sb 2 Te 3 , are novel quantum states of matter that can be generated by strong spin-orbit interaction and protected by time-reversal symmetry [1] , [2] , [3] , [4] , [5] . Study of TSSs provides us with unique opportunities to explore exotic physical phenomena such as spin Hall effects and topological phase transitions and a prospective materials base for construction of room-temperature quantum devices for spintronics and topological quantum computation [1] , [2] , [3] , [4] , [6] . Although ultrahigh-vacuum (UHV) surface probes such as scanning tunnelling microscopy (STM) [7] , [8] and angle-resolved photoemission spectroscopy (ARPES) [9] , [10] , [11] can identify individual TSSs, electrical [12] and optical [13] , [14] , [15] techniques to detect and control the TSSs in the ambient are essential to implement practical applications. So far, conventional transport and optical measurements have suffered from the simultaneous presence of bulk free-carrier states, quantum well states (QWSs) and TSSs in routinely prepared TI single crystals and thin films. The TSSs are distinguished from the bulk and QWSs by their unique topological origin. As routinely prepared TI single crystals and thin films are often unintentionally doped due to impurities or native defects, the nominally insulating bulk inevitably possesses free-carrier states that seriously affect standard transport and optical measurements. In addition, the QWSs, generated by band bending (or Se vacancies) near the surface, appear as discrete conducting states crossing the Fermi level E F , thereby adding to the conductance as measured by electrical and optical techniques. The simultaneous presence of TSSs, bulk free-carrier states and QWSs in general make it prohibitively difficult to selectively probe the TSSs, and so far only UHV surface probes such as STM and ARPES techniques were able to directly resolve individual TSSs in real and momentum spaces, respectively [7] , [9] . However, key physical properties such as transport and electromagnetic properties of TSSs are not readily accessible as the standard electrical and optical measurements yield the total response of TSSs, QWSs and bulk free-carrier states. Indeed, recent terahertz spectroscopic investigations on Bi 1.5 Sb 0.5 Te 1.8 Se 1.2 (BSTS) [16] and Bi 2 Se 3 (ref. 17 ) reported detection of the contributions from the TSSs, but unambiguously disentangling the individual contributions of constituent entities was so far not feasible due to various problems related to impurities, native defects and surface degradations. In fact, routinely prepared TI samples yield unreasonably large conductance values of the order of 10 −3 Ω −1 , almost 10 2 times the single conductance quantum G 0 = e 2 / h =3.97 × 10 −5 Ω −1 ( e electronic charge and h Planck’s constant), expected for an ideal TI surface. Even for TI films of thickness down to 10 quintuple layers (QL), presumably devoid of bulk free-carrier states, the reported conductance level is ~30 G 0 (refs 18 , 19 ). A proper means to selectively probe the TSSs would be highly desirable for further research on the dynamics of TSSs and their physical properties towards practical applications. Here, we show that the combination of terahertz time-domain spectroscopy (THz-TDS) and high-quality ultrathin TI films grown by molecular beam epitaxy (MBE) can successfully resolve this outstanding issue. We report on our THz-TDS study of a series of ultrathin Bi 2 Se 3 films grown by MBE, with which we track a series of topological phase transitions from the three-dimensional (3D) bulk topological insulator to the two-dimensional (2D) hybrid topological insulator (HTI) and then to the 2D trivial insulator as we vary the film thickness from 8 QL to 2 QL. For the thickness of 3 QL, corresponding to the HTI phase, we observe a terahertz conductance of 2 G 0 , namely, a single conductance quantum G 0 from each of the top and bottom surfaces of the TI film, the ultimate minimum conductance theoretically predicted [20] , [21] , [22] , [23] . This also leads to a quantized terahertz absorbance of 4 α ≈2.9% ( α the fine structure constant) for a pair of TSSs. In contrast, the 2 QL film exhibits vanishing conductance, consistent with the 2D trivial insulator phase. Also, the infrared-active in-plane phonon mode at 9 meV was found to be strongly coupled to the TSSs as evidenced by its asymmetric Fano-like lineshape. This interaction mechanism suggests an intriguing possibility to control the TSS dynamics through intentional modulation of the lattice. Our experiment demonstrates the feasibility to isolate, detect and manipulate TSSs in the ambient at room temperature for future fundamental research on the novel physics of TIs and their practical applications. 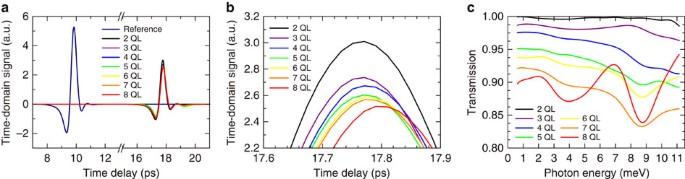Figure 1: Time-domain signal and transmission of a series of Bi2Se3thin films acquired at room temperature. (a) Time-domain picosecond (ps) pulses transmitted through vacuum (reference) and Bi2Se3thin films (2–8 QL) where 1 QL (quintuple layer) is 0.954 nm. (b) The sample pulse peaks are magnified. The systematic time delay and peak reduction relative to the reference pulse peak reflect the changes in both the film thickness and the terahertz conductivity. (c) Power transmission spectraTobtained from the Fourier transforms of the time-domain signals. Here,Tdecreases with increasing film thickness and exhibits free-carrier absorption in the d.c. limit, quantum well state (QWS) intersubband transitions around 4 meV, and an in-plane phonon mode around 9 meV. Terahertz conductivity spectra Our Bi 2 Se 3 thin films of 2, 3, 4, 5, 6, 7 and 8 QL thickness (1 QL=0.954 nm here) on Si (100) substrates were grown by MBE (see Methods, Supplementary Note 1 , Supplementary Figs 1–4 , and Supplementary Table 1 ). Their layer-by-layer growth was monitored in situ by reflection high-energy electron diffraction (RHEED). Our terahertz transmission measurements on the films were performed at room temperature within 30 min of their growth. Both the real part G 1 ( ω ) and the imaginary part G 2 ( ω ) of the complex conductance G ( ω ) of a given TI film were acquired as functions of angular frequency ω , independently and simultaneously from its measured (substrate-normalized) complex transmittance, , characterized by the power transmission T and the phase shift ϕ (see Methods). We present the measured conductance values in units of the conductance quantum G 0 . In particular, for a system with discrete (quantized) conducting channels, this representation is convenient for counting the number of individual conducting channels. Analysis of the low-frequency limit of the terahertz conductance spectrum provides us with an indirect, contact-free method to investigate the quasi-d.c. transport properties. Figure 1a shows the time-domain picosecond pulses transmitted through vacuum (reference) and our Bi 2 Se 3 thin films (2–8 QL) acquired at room temperature. Relative to the reference signal, the sample signals exhibit time delay and power absorption as a result of the film response. The systematic changes reflect both the thickness and the evolving terahertz spectral characteristics of our Bi 2 Se 3 films (an expanded view of the sample pulse peaks in Fig. 1b ). The amplitude and phase of the Fourier transforms of the time-domain signals are normalized against those of bare Si substrates to yield the power transmission T and the phase shift ϕ . The power transmission T ( Fig. 1c ) here decreases with increasing film thickness as also indicated by the peak reduction of the time-domain pulses. At the low-frequency end, T decreases in regular steps with the increasing number of QLs, as expected, except for a jump between 4 QL and 5 QL, before the bulk free-carrier states begin to enter systematically (as explained below). The power transmission also shows a strong dip centred around 9 meV and a broad depression around 4 meV, corresponding to the α phonon mode and the QWS intersubband transitions, respectively. Both features also change with film thickness in a remarkable manner. Figure 1: Time-domain signal and transmission of a series of Bi 2 Se 3 thin films acquired at room temperature. ( a ) Time-domain picosecond (ps) pulses transmitted through vacuum (reference) and Bi 2 Se 3 thin films (2–8 QL) where 1 QL (quintuple layer) is 0.954 nm. ( b ) The sample pulse peaks are magnified. The systematic time delay and peak reduction relative to the reference pulse peak reflect the changes in both the film thickness and the terahertz conductivity. ( c ) Power transmission spectra T obtained from the Fourier transforms of the time-domain signals. Here, T decreases with increasing film thickness and exhibits free-carrier absorption in the d.c. limit, quantum well state (QWS) intersubband transitions around 4 meV, and an in-plane phonon mode around 9 meV. Full size image In Fig. 2 , we show the real ( G 1 ) and the imaginary ( G 2 ) parts of the complex conductance ( G ) of our Bi 2 Se 3 series of thin films at room temperature. The conductance level observed in our TI films is much smaller than that reported for routinely prepared Bi 2 Se 3 films of comparable thickness by a factor of 30 at least [15] , which indicates that residual conductance due to the bulk free-carrier states has been minimized in our samples, with the corresponding Fermi level E F closer to the Dirac point in the midgap. The overall level of the real part G 1 systematically decreases with decreasing film thickness as expected, revealing a conspicuous evolution of key spectral features as well. We clearly identify three components in each G 1 spectrum: a weakly frequency-dependent conductance background at low frequencies seen below 2 meV, a broad absorption feature centred around 4 meV and a strong absorption peak located near 9 meV. The zero-frequency extrapolation of the nearly flat G 1 background should match the d.c. conductance values as measured by transport experiment. We note here that, in the ultrathin-film limit, standard transport measurements become unreliable due to the high sensitivity to the device geometry and the well-known difficulty associated with separating the TSS signal from the noisy background [18] . Indeed, our alternative terahertz technique provides us with much more reliable quasi-d.c. conductance values, which, in units of G 0 , are actually the total number of discrete (quantized) conducting channels contributed by TSSs and QWSs in the absence of bulk free-carrier states for sufficiently thin films. As the film thickness decreases from 8 QL to 2 QL, we expect both the bulk free-carrier states and QWSs to sequentially move away from the Fermi level, eventually leaving only a single TSS isolated on each of the top and bottom surfaces of our ultrathin TI films (the purple curve in Fig. 2a ). The low-frequency terahertz conductance displayed in Fig. 2a thus exhibits a monotonic decrease in line with such expectations. 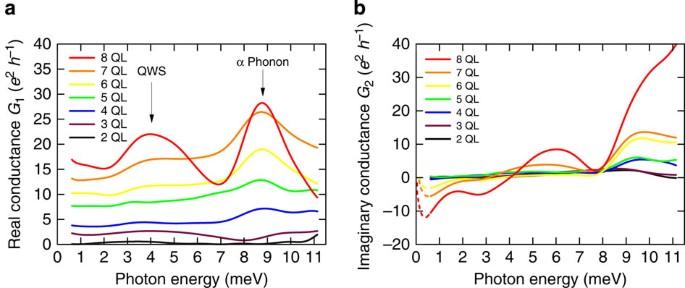Figure 2: Terahertz conductance spectra of a series of Bi2Se3thin films at room temperature. (a) The real part of the conductance spectraG1showing the predominant features at the low-energy end (free-carrier absorption), around 4 meV (quantum well state (QWS) intersubband transitions), and around 9 meV (the α phonon).G1is given in units of the conductance quantumG0=e2/h(eelectron charge andhPlanck’s constant). Here 1 QL (quintuple layer) is 0.954 nm. (b) The imaginary part of the conductance spectraG2reflecting the concomitant phase distortions due to the aforementioned features in (a).G2is also given in units ofG0. The broken lines indicateG2obtained by a linear extrapolation of the measured phase shiftϕtowards zero frequency. Figure 2b shows the imaginary part G 2 , the spectral shape of which clearly reflects the concomitant phase distortions mainly due to the two aforementioned absorption features observed around 4 and 9 meV. The broken lines indicate G 2 obtained by a linear extrapolation of the measured phase shift ϕ towards zero frequency, all of which converge towards zero as expected. However, the solid lines are not dependent on this extrapolation procedure as they have been determined frequency by frequency without resorting to a Kramers–Kronig analysis (see Methods). Figure 2: Terahertz conductance spectra of a series of Bi 2 Se 3 thin films at room temperature. ( a ) The real part of the conductance spectra G 1 showing the predominant features at the low-energy end (free-carrier absorption), around 4 meV (quantum well state (QWS) intersubband transitions), and around 9 meV (the α phonon). G 1 is given in units of the conductance quantum G 0 = e 2 / h ( e electron charge and h Planck’s constant). Here 1 QL (quintuple layer) is 0.954 nm. ( b ) The imaginary part of the conductance spectra G 2 reflecting the concomitant phase distortions due to the aforementioned features in ( a ). G 2 is also given in units of G 0 . The broken lines indicate G 2 obtained by a linear extrapolation of the measured phase shift ϕ towards zero frequency. Full size image Isolation of TSSs and topological phase transitions We show the evolving band structure of our Bi 2 Se 3 films as a function of thickness in Fig. 3a and the concomitant increase in the d.c.-limit conductance, G 1 ( ω →0), in units of the conductance quantum G 0 , in Fig. 3b . As the film thickness increases from 2 QL to 8 QL, we see TSSs, QWSs and bulk free-carrier states appear in sequence, manifested by their individual conductance contributions. In the 2 QL film, the d.c.-limit real conductance was essentially zero within our experimental accuracy ( Figs 2a , 3b ). The 2 QL film, during its MBE growth, did exhibit clear RHEED patterns, confirming proper formation of well-defined unit-cell layers. Furthermore, we still see phonon absorption features around 10 meV even in this ultrathin film ( Fig. 2a ). These observations strongly suggest that the 2 QL film actually belongs to the 2D trivial insulator phase. As the film thickness increases, one expects to encounter a topologically-nontrivial 2D insulator phase (quantum spin Hall phase). Indeed, theoretical calculations [20] , [21] show that a TI film will alternate between these two phases, in an oscillatory manner, as a function of thickness as the Chern number of the surface bands changes, signalling the first topological phase transition with the band inversion at the critical thickness of 2.5 nm (1 QL≈1 nm). This critical thickness lies between 2 QL and 3 QL for the present case of Bi 2 Se 3 . In this scenario, the 3 QL film naturally corresponds to the topologically nontrivial 2D insulator phase, naturally with its d.c. conductance of 2 G 0 , consistent with our experiment, that is, with one conductance quantum contributed by a TSS on each of the two surfaces. For this case of 3 QL, the TSSs on top and bottom surfaces are quantum mechanically coupled, hybridizing with each other as the wave function from one surface penetrates into the other (their evanescent tails about 3 QL≈3 nm long) [15] , [20] , [21] , and the usual Dirac cone now turns into a pair of Dirac hyperbolas (in the E versus k space). The implication for the experimental data is that now coherent backscattering becomes possible as a forward-moving, up-spin state on the top surface can bounce back into a backward-moving, up-spin state on the bottom surface. Such a newly formed spin-conserving scattering channel increases the scattering rate, as confirmed by its four-fold increase compared with the 8 QL case in which the two TSSs are decoupled ( Fig. 4c ). One can think of the 3 QL film as forming a 2D HTI. In this context, the four-band effective model for Bi 2 Se 3 (ref. 22 ) was shown to be essentially equivalent to the 2D quantum spin Hall effective Hamiltonian [23] , applicable to HgTe quantum wells [20] , [24] . 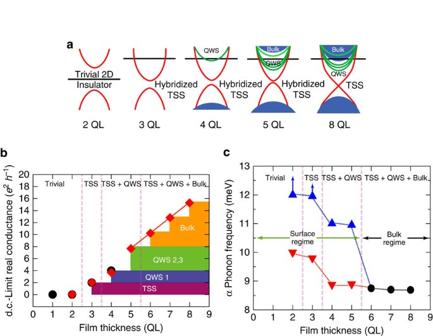Figure 3: Evolving band structure of Bi2Se3ultrathin films with their d.c.-limit real conductance andαphonon frequencies. (a) Band diagrams for the various phases of Bi2Se3ultrathin films schematically representing the Fermi level (black line), the topological surface states (TSSs) (red curve), the quantum well states (QWSs) (green curve) and the bulk free-carrier states (blue region). Here 1 QL (quintuple layer) is 0.954 nm. The theory in refs20,21,22,23predicts that, below 3 QL, the film is a trivial 2D insulator and that the 3-QL film is a 2D hybrid topological insulator. The 4-QL and 5-QL films admit a single QWS and triple QWSs. Beyond 5 QL, the bulk free-carrier states also cross the Fermi level. In the 8-QL film, the TSSs on the top and bottom surfaces decouple, and the linear dispersion is restored. (b) The d.c.-limit real conductance of Bi2Se3ultrathin films in units of the conductance quantumG0=e2/h(eelectron charge andhPlanck’s constant). Black circles indicate theory (refs20,21,22,23for 1–3 QL and ref.27for 4 QL). Red diamonds represent our experiment. QWS 1 and QWS 2, 3 represent the conductance contributions of the first (4 QL) and second (5 QL) groups of QWSs. The broken vertical lines mark the sequential emergence of TSS, QWS and bulk free-carrier states. The red line is the least-square fit to the data points for 5–8 QL, whose slope yields 2.5G0/QL=1.01 × 103Ω−1cm−1, consistent with the bulk conductivity reported in ref.13. (c) Theαphonon frequencies of the intrinsic mode around 9 meV (black circles and red triangles) and the higher-lying extrinsic mode induced by a finite-size effect for the films of thickness 5 QL and lower (blue triangles). For the 3-QL and 2-QL films, the higher-lying extrinsic mode lies just outside our measurement range and the lower limit was determined from a two-Lorentz fit (blue arrows). The mode splitting is observed in the surface regime (5 QL and lower, green arrows) but not in the bulk regime (6 QL and higher, black arrows). Figure 3: Evolving band structure of Bi 2 Se 3 ultrathin films with their d.c.-limit real conductance and α phonon frequencies. ( a ) Band diagrams for the various phases of Bi 2 Se 3 ultrathin films schematically representing the Fermi level (black line), the topological surface states (TSSs) (red curve), the quantum well states (QWSs) (green curve) and the bulk free-carrier states (blue region). Here 1 QL (quintuple layer) is 0.954 nm. The theory in refs 20 , 21 , 22 , 23 predicts that, below 3 QL, the film is a trivial 2D insulator and that the 3-QL film is a 2D hybrid topological insulator. The 4-QL and 5-QL films admit a single QWS and triple QWSs. Beyond 5 QL, the bulk free-carrier states also cross the Fermi level. In the 8-QL film, the TSSs on the top and bottom surfaces decouple, and the linear dispersion is restored. ( b ) The d.c.-limit real conductance of Bi 2 Se 3 ultrathin films in units of the conductance quantum G 0 = e 2 / h ( e electron charge and h Planck’s constant). Black circles indicate theory (refs 20 , 21 , 22 , 23 for 1–3 QL and ref. 27 for 4 QL). Red diamonds represent our experiment. QWS 1 and QWS 2, 3 represent the conductance contributions of the first (4 QL) and second (5 QL) groups of QWSs. The broken vertical lines mark the sequential emergence of TSS, QWS and bulk free-carrier states. The red line is the least-square fit to the data points for 5–8 QL, whose slope yields 2.5 G 0 /QL=1.01 × 10 3 Ω −1 cm −1 , consistent with the bulk conductivity reported in ref. 13 . ( c ) The α phonon frequencies of the intrinsic mode around 9 meV (black circles and red triangles) and the higher-lying extrinsic mode induced by a finite-size effect for the films of thickness 5 QL and lower (blue triangles). For the 3-QL and 2-QL films, the higher-lying extrinsic mode lies just outside our measurement range and the lower limit was determined from a two-Lorentz fit (blue arrows). The mode splitting is observed in the surface regime (5 QL and lower, green arrows) but not in the bulk regime (6 QL and higher, black arrows). 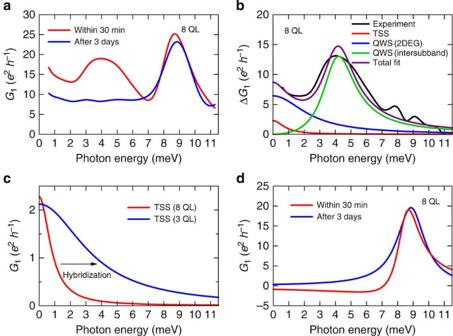Figure 4: Ageing-effect study of a Bi2Se3film of 8 quintuple layer thickness. (a) The real conductance spectraG1of our 8-QL (quintuple layer) Bi2Se3film measured within 30 min (red) and after 3 days (blue) of its growth.G1is given in units of the conductance quantumG0=e2/h(eelectron charge andhPlanck’s constant). (b) The difference conductance ΔG1, lost by surface degradation, fitted to a Drude–Lorentz model. The topological surface state (TSS) component (red) here can be essentially extracted from the low-energy part of ΔG1. The quantum well state (QWS) consists of the Drude component (blue) representing a two-dimensional electron gas (2DEG) and the Lorentzian component (green) of intersubband transitions. The total fit (purple) is compared with experiment (black). (c) The Drude components representing the contribution of the two Dirac cones (red) on the top and bottom surfaces of the 8-QL film, and that of the two Dirac hyperbola pairs (blue) likewise from the 3-QL film (obtained by a separate Drude–Lorentz fit). The scattering rate (the linewidth ofG1) has increased by a factor of 4 due to the surface hybridization in the 2D hybrid topological insulator phase prevalent in the 3-QL film. (d) Theαphonon lineshape representing electron–phonon coupling strength, asymmetric (Fano-like) before ageing (red, within 30 min) and symmetric (Lorentzian) after ageing (blue, after 3 days). On ageing, the Fano parameter 1/qhas been reduced by a factor of 20 and its sign has reversed (from +0.29 to −0.014), probably due to the destruction of the TSSs. Full size image Figure 4: Ageing-effect study of a Bi 2 Se 3 film of 8 quintuple layer thickness. ( a ) The real conductance spectra G 1 of our 8-QL (quintuple layer) Bi 2 Se 3 film measured within 30 min (red) and after 3 days (blue) of its growth. G 1 is given in units of the conductance quantum G 0 = e 2 / h ( e electron charge and h Planck’s constant). ( b ) The difference conductance Δ G 1 , lost by surface degradation, fitted to a Drude–Lorentz model. The topological surface state (TSS) component (red) here can be essentially extracted from the low-energy part of Δ G 1 . The quantum well state (QWS) consists of the Drude component (blue) representing a two-dimensional electron gas (2DEG) and the Lorentzian component (green) of intersubband transitions. The total fit (purple) is compared with experiment (black). ( c ) The Drude components representing the contribution of the two Dirac cones (red) on the top and bottom surfaces of the 8-QL film, and that of the two Dirac hyperbola pairs (blue) likewise from the 3-QL film (obtained by a separate Drude–Lorentz fit). The scattering rate (the linewidth of G 1 ) has increased by a factor of 4 due to the surface hybridization in the 2D hybrid topological insulator phase prevalent in the 3-QL film. ( d ) The α phonon lineshape representing electron–phonon coupling strength, asymmetric (Fano-like) before ageing (red, within 30 min) and symmetric (Lorentzian) after ageing (blue, after 3 days). On ageing, the Fano parameter 1/ q has been reduced by a factor of 20 and its sign has reversed (from +0.29 to −0.014), probably due to the destruction of the TSSs. Full size image Universal terahertz absorption by TSSs Interestingly, the single conductance quantum associated with a single TSS leads to a universal terahertz absorbance of 4 α ≈0.29% for a pair of TSSs in the case of a freestanding 3 QL-thick Bi 2 Se 3 film ( α ≡ e 2 / ħc ≈1/137 is the fine structure constant, ħ ≡ h /2 π is the reduced Planck’s constant and c is the speed of light in vacuum). For graphene, the quantized optical absorption due to the interband transition in the visible range was theoretically proposed and experimentally confirmed [25] . Without many-body effects, this universal optical absorption by a graphene monolayer is simply given by For TIs, we propose here a new universal terahertz absorption of 4 α associated with the intraband absorption by a pair of TSSs (one TSS per surface). In general, the transmission T f of an ultrathin film can be obtained with Tinkham’s formula [26] , according to which T f of an ultrathin TI film is given by the second equality valid for a small value of Z 0 G 0 /( η s +1) where G =2 G 0 is the conductance of the TSS pair, Z 0 =4 π / c is the vacuum impedance, G 0 = e 2 / h is the conductance quantum and η s is the substrate refractive index (3.414 for Si). Equation (2) is valid under the two conditions: the film thickness is much smaller than the wavelength, and the film conductivity is much higher than that of the substrate. The first condition is based on the small (radian) value of wavenumber times thickness, which, in our case, is (conservatively estimating) 100 cm −1 × 10 nm=10 −4 compared with, for example, π . As to the second condition, our substrate conductivity is only of the order of 0.1 Ω −1 cm −1 , much smaller than the order of G 0 /QL=400 Ω −1 cm −1 for the film conductivity. The intraband absorption A f for a pair of TSSs can be then written as At the low-frequency end, our terahertz measurements yield a very close value of A f =0.0134, extracted from the transmission T f of our 3 QL film possessing only a pair of TSSs as its only low-frequency absorption channel. For a freestanding ultrathin TI film (with η s =1 for vacuum), we will have a universal terahertz absorption of which is slightly larger than the universal optical absorption of πα ≈2.3% for graphene. Systematic entry of QWSs and bulk free-carrier states For the 4 QL film, an additional conductance of 2 G 0 enters the system, again presumably G 0 from each surface. We can unambiguously assign this change to the entry of a single QWS based on a simple model ( Supplementary Note 2 ) as suggested by the tight binding model calculation in ref. 27 and by previous ARPES reports [9] , [11] . For the 4 QL film, the surface quantum wells generated by band bending (or Se vacancies) near the surface become deep enough to sustain a well-defined eigenstate that crosses the Fermi level. For the 5 QL Bi 2 Se 3 film, we estimate that the quantum wells on both surfaces hold three eigenstates each and together contribute 6 G 0 overall as confirmed by our data ( Fig. 3b ). We note that, for a 5 QL Bi 2 Se 3 film, previous ARPES experiment clearly showed the presence of two QWSs crossing the Fermi level with the bulk band at least 100 meV above the Fermi level [9] . For the thickness range of 6 QL and higher, the additional conductance comes from the bulk free-carrier states, with the lowest point of the conduction band now touching the Fermi level. In contrast, for sufficiently thin films, these bulk free-carrier states are pushed away from the Fermi level and do not contribute any conductance as detected by transport and optical measurements. The conductance from the bulk free-carrier states exhibits a linear correlation with the film thickness; beyond 5 QL, a new QL contributes a constant conductance of about 2.5 G 0 ( Fig. 3b ). Well into the thick-film regime, the d.c.-limit real conductance should be essentially proportional to the film thickness. The slope of the straight line least-square fitted to the last four data points for our 5–8 QL films ( Fig. 3b ) therefore indicates that we now enter the bulk regime and that the bulk conductivity is 2.5 G 0 /QL=1.01 × 10 3 Ω −1 cm −1 , which is consistent with the bulk conductivity value of ~1 × 10 3 Ω −1 cm −1 extracted from the single-crystal study reported in ref. 13 . We next return to the strong absorption feature around 9 meV in the real conductance ( G 1 ) spectra ( Fig. 2a ) due to the infrared-active in-plane phonon mode with E u symmetry (called the α phonon mode). This phonon mode exhibits an asymmetric lineshape and a spectral weight roughly proportional to the number of QLs, but its oscillator strength is significantly enhanced far beyond theoretical estimation [28] . The α phonon in our spectra and the higher-frequency β phonon at around 16 meV (not shown) as reported in the literature were predicted to have comparable spectral weights, but the α phonon mode exhibits an oscillator strength much greater than that reported for the β phonon mode, as measured by infrared spectroscopy [13] . Figure 3c presents the centre frequency of the α phonon in our Bi 2 Se 3 thin films as a function of film thickness. In the bulk regime (6 QL and higher), the centre frequency is more or less constant, whereas, into the surface regime (5 QL and lower), a second, higher-lying phonon mode emerges at ~11 meV ( Fig. 2a ). For the 3 QL and 2 QL films, this mode lies just outside our measurement range, and its centre frequency was determined from a two-Lorentz fit. The two-mode behaviour can be explained in terms of a finite-size effect. As we go into the ultrathin-film limit, the strength of the new extrinsic (surface-like) α phonon mode, essentially confined to the film-substrate interface (with a higher resonance frequency), becomes comparable to that of the intrinsic (bulk-like) α phonon mode. This surface-like mode emerges as a result of interaction between the innermost QL and the Si substrate. For the 1,590 cm −1 in-plane phonon mode in bilayer graphene, a similar mode splitting due to broken inversion symmetry (the presence of substrate potential) was observed [29] . The present mode splitting can be explained by a classical model employing two oscillators coupled by a weak interlayer van der Waals interaction [30] . In the weak-coupling limit, only one of the two initially degenerate eigenfrequencies blueshifts while the other essentially retains the original resonance frequency of the two identical, uncoupled oscillators. This intermode coupling is sufficiently screened by the bulk free-carrier states in the bulk regime (6 QL and higher), but, for the surface regime (5 QL and lower), the interlayer coupling increases as the bulk free-carrier states disappear and as the TSSs on the top and bottom surfaces hybridize. Below 3 QL, both the lower- and higher-lying modes exhibit blue shifts most likely due to enhanced van der Waals coupling [31] between them. Decoupled TSSs and strong phonon coupling We now discuss the broad absorption feature around 4 meV ( Figs 2a , 4a ) in the real conductance G 1 spectra of our Bi 2 Se 3 thin films. This peak is most intense in the 8 QL film and gradually weakens as the film thickness decreases ( Fig. 2a ). The energy scale of this mode is in good agreement with that of the intersubband transitions associated with the QWSs [11] . The QWSs have so far been directly observed only in Bi 2 Se 3 with in situ ARPES but not in any other TIs or by any other measurement methods, presumably due to either surface contamination or residual doping [11] . Figure 4a shows the real conductance G 1 spectra of our 8 QL Bi 2 Se 3 film measured within 30 min and after 3 days of its growth. While the α phonon mode changed in a subtle manner, the QWS peak completely vanished, leaving behind only the broad Drude-like background coming from the bulk free-carrier states. The lost spectral weight of 8 G 0 represents the contributions of the surface states, namely, the QWSs constituting a two-dimensional electron gas (2DEG) and the TSSs confined to the top and bottom surfaces. Similar degradations were observed in all other films regardless of their thickness, especially even in those films in the surface regime (5 QL and below) in which the bulk free-carrier state contributions are absent [32] . This ageing-effect study provides us with an unexpected opportunity to selectively probe the TSSs and QWSs formed on fresh TI surfaces. Figure 4b shows Δ G 1 ( ω ), the real conductance associated with the lost TSSs and QWS states for the 8 QL film, obtained from the spectra in Fig. 4a by subtraction, now fitted to a Drude–Lorentz model. The detailed results are given in Tables 1 and 2 and Methods. We have extracted the per-channel (per-surface) areal electron densities of n 2D (TSS)=8.40 × 10 10 cm −2 and n 2D (QWS)=4.50 × 10 12 cm −2 and the mobilities of μ (TSS)=2,880 cm 2 V −1 s −1 and μ (QWS)=54 cm 2 V −1 s −1 , all of which agree well with the literature values [12] , [18] . Here, we employed the effective masses of m *=0.07 m e for the TSS on the Dirac cones and m *=0.15 m e for the QWS comprising the 2DEG states (both estimated at E F ) obtained from Hall measurements [33] , [34] . We compare in Fig. 4c the real conductance G 1 spectra for the two hybridized TSSs in the 3 QL film with that for the uncoupled TSSs in the 8 QL film. In contrast to the case of Dirac-conic electrons (8 QL), the coherent backscattering is enhanced for Dirac-hyperbolic electrons (3 QL) [15] , leading to an increased scattering rate and hence a broadened linewidth of G 1 in the 3 QL case, as shown in Fig. 4c . Table 1 Free-carrier parameters for a 8-QL Bi 2 Se 3 film. Full size table Table 2 QWS intersubband and α phonon parameters. Full size table The subtle changes in the α phonon mode on surface degradation supply a critical piece of information on the electron–phonon interaction in Bi 2 Se 3 . For the 8 QL film, we have fitted the α phonon lineshape to a Fano model, extracting the Fano parameter q before and after surface degradation ( Fig. 4d ). The Fano-fit details are given in Table 2 and Supplementary Note 3 . The magnitude of 1/ q , proportional to the electron–phonon coupling strength, controls the degree of lineshape distortion away from the symmetric Lorentzian, while its sign change reflects the phase difference between the counterpart electron wave functions before and after the surface degradation. The asymmetry parameter 1/ q =+0.29 extracted from the fresh 8 QL film agrees with that of the Raman-active phonon mode located at 70 cm −1 , both in magnitude (within a factor of 3) and in sign [35] . In contrast, the magnitude of 1/ q =−0.014 extracted after ageing is smaller by a factor of 20 and its sign has reversed. For the fresh film (within 30 min of growth), the asymmetry is characterized by a down-shift of the low-energy tail and an up-shift of the high-energy tail, but an opposite trend has been noted in the degraded film (after 3 days of growth). Without an obvious way to obtain a π phase shift from the phonon mode alone, the sign reversal should be attributed to an electron continuum coupled to the phonon system, that is, the surface states destroyed by the surface degradation ( Supplementary Note 3 and Supplementary Fig. 5 ). Further, although the degradation of QWS (2DEG) probably affects the magnitude of the Fano parameter q , the critical sign change is most likely to be associated with the destruction of the TSSs [36] . Our analysis opens up a way to check the presence and absence of TSSs and hence the topological character of TI surfaces in the ambient at room temperature through a relatively simple phonon analysis based on standard THz-TDS. The versatile role played by the terahertz spectroscopic technique in elucidating the rich physics of TIs as revealed here will potentially open up many fascinating possibilities. The TSSs directly couple with terahertz radiation with their characteristic energy scale naturally falling into the subterahertz frequency range, suggesting at the same time many novel terahertz device applications. In view of present difficulties associated with standard transport measurements, terahertz techniques will provide a useful tool to study TIs in a nondestructive and contact-free manner. As the infrared-active phonon modes in TIs directly couple with the terahertz radiation as well, the strong TSS–phonon coupling will enable us to control the TSSs by manipulating the lattice with, for example, powerful terahertz pulses, possibly leading to terahertz photonics or plasmonics applications. Overall, the intriguing combination of TIs and THz-TDS as adopted in the present study to detect and utilize the novel TSSs will play a critical role in developing tangible future applications in practical room-temperature quantum devices. MBE thin-film growth As Se- and Te-based chalcogenide compounds have a layered crystal structure, a method employing homogeneously interdiffused atomic layers can be used to fabricate a high-quality layered crystal structure (refs 37 , 38 , 39 ). The self-ordering process for single-crystalline Bi 2 Se 3 films through short-range diffusion that can overcome the synthetic limitations of slow diffusion rates in solid-state reactions requires the formation of alternate layers of Bi atoms and a high level of excess Se atoms. During this process, each atomically controlled layer diffuses into its adjacent layers and forms a well-ordered crystalline structure. For the present study, thin films of the starting composition of [(Bi(0.486 nm)Se(1.846 nm))] n (where n is to be the total number of unit-cell layers) were initially grown on Si (100) substrates by the thermal evaporation method, as each layer was controlled independently within 1 nm thickness. The deposition process involves individually operating source shutters combined with a quartz crystal monitor. As-grown films were annealed in situ at 200 °C for 20 min under a vacuum of 10 −8 Torr. The surface roughness and density of each deposited elemental layer were confirmed by X-ray reflectivity measurements. Also, the total thickness and composition ratio of the final layer-by-layer grown films were measured using X-ray reflectivity, Rutherford backscattering spectroscopy and inductively coupled plasma optical-emission spectrometry, as shown in Supplementary Note 1 . We exclude the 1 QL film from our study as it did not form properly during its growth as revealed by its diffuse RHEED pattern. Terahertz time-domain spectroscopy Terahertz spectroscopy probes the electromagnetic response of material media ranging from metals to semiconductors to insulators typically in the frequency range of 0.1–3 THz (3–100 cm −1 or 0.5–12 meV). The primary responses come from free carriers and lattice vibrations in accordance with their characteristic energy scales. In the present case, the free carriers in bulk states, TSSs and QWSs directly couple with the terahertz radiation and exhibit distinctive absorption features within our experimental frequency range. The bulk free-carrier states and the TSSs exhibit Drude-like conductance spectra, revealing key electronic parameters such as the carrier density, the effective mass and the scattering rate. In addition, subtle changes in the resonance frequency, the oscillator strength and the lineshape (possibly including Fano distortions) of the phonon modes in connection with their interaction with TSSs and QWSs are reflected in the terahertz absorption spectra. We conducted our terahertz measurements with a TeraView TPS 3000 Spectrometer, utilizing picosecond pulses in the time domain to acquire the complex transmittance through our Bi 2 Se 3 ultrathin films. Normalization against the substrate response is achieved by a separate measurement on a blank substrate. Internal reflections within the substrate that usually result in interference fringes were removed in the time domain by limiting the measurement time-window to retain only the primary pulse through the sample. Time-domain signals are then Fourier-transformed to generate frequency-dependent spectral functions (see Supplementary Note 4 and Supplementary Fig. 6 for discussion on the accuracy of our terahertz spectroscopic method). The normalized complex transmittance is then converted into the complex conductance spectra based on Tinkham’s formula [26] , valid in the ultrathin-film limit as studied here. The formula is given by t fs / t s =1/[1+ Z 0 G /( η s +1)] where t fs and t s are the complex transmission coefficients of the sample (film plus substrate) and the bare substrate, respectively, while Z 0 is the vacuum impedance, G the conductance of the film and η s the refractive index of the bare substrate. For bulk free-carrier states, G = σd where σ is the optical conductivity and d is the thickness of the film. Extraction of TSS and QWS characteristic parameters We employed a Drude–Lorentz model to fit the surface conductivity σ surf ( ω ) as well as the bulk conductivity σ bulk ( ω ) spectra of our Bi 2 Se 3 thin films: where ω p, TSS ( ω p,QWS ) and γ TSS ( γ QWS ) are the plasma frequency and scattering rate, respectively, for the TSSs (QWSs) while Ω p,QWS , Ω 0,QWS , and Γ QWS are the oscillator strength, centre frequency and damping rate, respectively, for the QWS intersubband transitions; where ω p,bulk and γ bulk are the plasma frequency and scattering rate, respectively, for the bulk free-carrier states while Ω p,ph , Ω 0,ph and Γ ph are the oscillator strength, centre frequency and damping rate, respectively, for the α phonon. The constant L ∞ ≡(1– ε ∞ )/4 π is related to the background dielectric constant ε ∞ . Depending on film thickness, certain Drude terms could be absent. For example, for our 3 QL film, the Drude contribution comes solely from the TSSs. For the α phonon, we used an asymmetric Lorentzian for the films of thickness 6 QL and higher ( Supplementary Note 3 ) and two Lorentzian terms for those of thickness 5 QL and lower. The surface (TSS and QWS) and bulk (free carrier and α phonon) conductivities are separately multiplied by their corresponding thickness values and then added to match our conductance data G ( ω ): The surface thickness value d surf was taken to be 2.9 nm (refs 9 , 18 , 21 ), while the bulk thickness value d bulk was obtained from the number of QLs where 1 QL=0.954 nm (from Supplementary Fig. 2b ). Our ageing-effect study, described in the main text, enables us to remove the bulk free-carrier component of the terahertz conductance and thus to extract the key parameters associated with the TSSs and QWSs. Here we choose the 8-QL film and compare the terahertz spectra acquired within 30 min and after 2 weeks of its growth. Our 8-QL film initially contained the Drude contributions from the TSSs, QWSs (2DEG) and bulk free-carrier, while only the bulk free-carrier component remains after ageing. By taking the difference spectrum Δ G 1 , we isolate the contributions of TSSs and QWSs (2DEG) that disappear as a result of ageing. Therefore, Δ G 1 ( Fig. 4b ) contains just the TSSs and QWSs (2DEG), which can be readily separated due the substantial differences in their d.c.-limit real conductances and scattering rates. For our 3-QL film, the Drude contribution solely comes from the TSSs, with a four-fold increase in the scattering rate (due to hybridization) compared with the 8-QL case. The sheet carrier density n 2D for the TSSs (QWSs) is extracted from the plasma frequency determined from the aforementioned fit where m * is the electron effective mass, e is the electronic charge and ε 0 is the free-space permittivity. We find where c is the speed of light in vacuum. Here, we employed the effective masses of m *(TSS)=0.07 m e and m *(QWS)=0.15 m e (estimated at the Fermi level E F , m e electronic mass) obtained from previously reported Hall measurements [33] , [34] . The mobilities μ are obtained from the d.c. surface conductance G surf where G surf = σ surf ( ω →0) d surf = n 2D eμ and G surf = G 0 per TSS and per QWS: Our data set also yields the Fermi velocity of v F (TSS)=1.0 × 10 6 m s −1 . We employed here two standard relations: and m *(TSS)= ħk F / v F where k F is the Fermi wave vector. The Fermi velocity v F was calculated with n 2D (TSS) extracted from our experimental data and m *(TSS) obtained from the literature [33] . Our results are in good agreement with previous theoretical and experimental reports [12] , [22] . How to cite this article: Park, B. C. et al . Terahertz single conductance quantum and topological phase transitions in topological insulator Bi 2 Se 3 ultrathin films. Nat. Commun . 6:6552 doi: 10.1038/ncomms7552 (2015).